Gene copy number is differentially regulated in a multipartite virus Multipartite viruses have a genome divided into several nucleic acid segments, each encapsidated separately. An evident cost for these viral systems, particularly if some segments are rare, is the difficulty of gathering one copy of each segment to ensure infection. Here, we investigate the segment frequency-related cost by monitoring the copy number of the eight single-gene segments composing the genome of a plant nanovirus. We show that some viral genes accumulate at low frequency, whereas others dominate. We further show that the relative frequency of viral genes impacts both viral accumulation and symptom expression, and changes specifically in different hosts. Earlier proposed benefits of viral genome segmentation do not depend on the segments’ frequency and cannot explain our observations. We propose that the differential control of gene/segment copy number may represent an unforeseen benefit for multipartite viruses, which may compensate for the extra costs induced by the low-frequency segments. Viruses exhibit a wide diversity of genome organizations, mechanisms of replication and gene expression strategies. Viral genomes can be composed of single- or double-stranded molecules of RNA or DNA, expressing genes from mono- or polycistronic mRNAs, which can be sub-genomic or full-genome-length mRNAs. Within this diversity, the so-called segmented viruses—DNA or RNA viruses infecting bacteria, animals or plants [1] —have a genome composed of more than one nucleic acid molecule, with 2 to 12 genome segments depending on the viral species. Among the segmented viruses, the most puzzling biological systems are found in the multipartite viruses [2] (described in plants and fungi), where the genome segments are not co-packaged in a single viral particle but are encapsidated individually, forming an ensemble of particles that must be transmitted together in order to infect new cells. The functioning of these biological systems has long intrigued virologists and evolutionary biologists, who have striven to understand how such systems have evolved by modelling the parametric space in which the cost/benefit ratio is positive. Proposed advantages of genome compartmentalization are greater stability of smaller-sized segments [3] , a potential faster replication of small genomic segments [4] , or the increased genome shuffling that could result from genome segmentation and ‘multipartitism’ [5] , [6] , [7] , [8] , [9] , [10] . An obvious cost to genome compartmentalization is the necessity to either package together all segments, for segmented viruses, or to ensure the co-entry of an ensemble of virus particles containing at least one copy of each genomic segment [3] , [6] , [11] , for multipartite viruses. This cost increases dramatically with the number of segments constituting the viral genome, as amply discussed in the related literature, and recently reinvestigated in a theoretical study [12] . One aspect of multipartite virus biology that has not been investigated, empirically or theoretically, is the potential regulation of the relative frequencies of different genome segments. Indeed, all else being equal, the probability of infecting a host cell successfully, that is, the probability that all genome segments are transmitted in at least one copy, would be maximized if all segments occurred at equal frequency; deviations from this situation would increase the cost of genome compartmentalization. To address this knowledge gap, we tested whether the predicted situation of minimum cost is indeed observed in populations of the multipartite Faba bean necrotic stunt virus (FBNSV), or whether additional unknown constraints drive the frequency of different segments to different values. FBNSV is a member of the genus Nanovirus in the family Nanoviridae [2] . The FBNSV genome is composed of eight circular single-stranded DNA molecules of about 1 kb (segments C, M, N, R, S, U1, U2 and U4), each encoding a single gene and encapsidated separately [13] . The genome organization and function of each gene have been discussed previously in detail [13] , [14] . Briefly, C encodes a protein that interferes with the cell cycle and is a general enhancer of DNA replication; M produces the movement protein allowing viral cell-to-cell and long-distance transport within host plants; N encodes a nucleo-cytoplasmic shuttle protein of unknown biological function; R encodes the protein that governs replication of all viral genome segments by an unknown cellular DNA polymerase; S encodes the capsid protein encapsidating the different viral genome segments individually; Finally, U1, U2 and U4 encode proteins of unknown function. The infection of host plants by FBNSV as well as by other nanoviruses is restricted to phloem tissues and, because the coat protein appears mandatory for intra-plant movement [14] , it is generally assumed that individual segments move in the form of virus particles throughout the plant vasculature. In many host plants, member species of the genus Nanovirus induce severe stunting, often totally inhibiting further plant growth [15] . Here we report monitoring of the relative frequency of the eight single-gene-encoding segments constituting the genome of FBNSV during infection of host plants. We show that the various genes accumulate with very different frequencies within individual host plants. Moreover, starting from distinct inoculation conditions and relative segment frequencies, the viral system reproducibly reaches a comparable state, designated the ‘setpoint genome formula’, where each genome segment (or gene) accumulates to its specific relative frequency. Our results further suggest that the setpoint genome formula corresponds to a state resulting in increased viral accumulation and enhanced symptoms for the FBNSV system. Finally, we show that the FBNSV genome formula reaches a different setpoint in distinct host plant species. Our results hence indicate that multipartite viruses can differentially control the copy number of their different genes (or segments). We propose that this is an unforeseen potential benefit for multipartite viruses. Defining the genome formula of FBNSV A set of 50 Vicia faba plants was agro-inoculated with equal amounts of each of the eight genomic segments of the FBNSV genome [13] . The frequency of each segment, relative to total viral DNA, was estimated in the uppermost leaf of each plant by real-time quantitative PCR (Q-PCR) ~4 weeks post-infection, when the infection had fully developed and arrested further development of the plant. In three independent experimental replicates, despite a large variance between individual plants, each segment accumulated reproducibly at a specific median frequency ( Fig. 1 and Supplementary Table S1 ), which ranged from ~2 to 30% (segments S and U4, respectively). 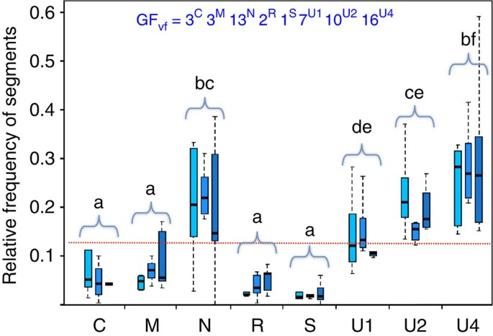Figure 1: The genome formula of FBNSV. The relative frequency of each genome segment of FBNSV was evaluated by Q-PCR in systemically infected leaves ofV. faba(Vf). The name of each segment is indicated below the graph. Results from three-independent replicates, named Vf-Agr1, Vf-Agr2 and Vf-Agr3, are plotted from left to right (with increasing shades of blue) for each segment. The number (n) of plants successfully infected and analysed in each of these three replicates isn=6,n=8 andn=5, respectively. The horizontal black bar within box-plots represents the median value of the distribution, and the vertical dotted line delineates 1.5 times the distance between the 25th and 75th percentile of the distribution. The dotted red line indicates the frequency at which all segments were agro-inoculated initially. There is no significant difference in the frequency of the segments between replicates (analysis of variance (ANOVA) test for the effect of the experiment replicates on the segment frequency:F2, 140=0.03,P-value=0.97). In contrast, differences between segments were highly significant (ANOVA test for the effect of the nature of the segment on its relative frequency,F7, 140=30.7,P-value<2 e-16). Significant differences in segment accumulation are indicated by letters and were assessed by Tukey HSD pair tests (allP-values are given in theSupplementary Table S1). The genome formula of FBNSV inV. faba, noted GFVfabove the graph, was calculated with the data pooled from Vf-Agr1-3. Figure 1: The genome formula of FBNSV. The relative frequency of each genome segment of FBNSV was evaluated by Q-PCR in systemically infected leaves of V. faba (Vf). The name of each segment is indicated below the graph. Results from three-independent replicates, named Vf-Agr1, Vf-Agr2 and Vf-Agr3, are plotted from left to right (with increasing shades of blue) for each segment. The number ( n ) of plants successfully infected and analysed in each of these three replicates is n =6, n =8 and n =5, respectively. The horizontal black bar within box-plots represents the median value of the distribution, and the vertical dotted line delineates 1.5 times the distance between the 25th and 75th percentile of the distribution. The dotted red line indicates the frequency at which all segments were agro-inoculated initially. There is no significant difference in the frequency of the segments between replicates (analysis of variance (ANOVA) test for the effect of the experiment replicates on the segment frequency: F 2, 140 =0.03, P -value=0.97). In contrast, differences between segments were highly significant (ANOVA test for the effect of the nature of the segment on its relative frequency, F 7, 140 =30.7, P -value<2 e-16). Significant differences in segment accumulation are indicated by letters and were assessed by Tukey HSD pair tests (all P -values are given in the Supplementary Table S1 ). The genome formula of FBNSV in V. faba , noted GF Vf above the graph, was calculated with the data pooled from Vf-Agr1-3. Full size image The reproducible accumulation of specific relative copy numbers for different viral genes poses the question of how best to describe the genome of a multipartite virus during infection of its host. To propose an easy and biologically sound description, and for practical use in this report, we define the term ‘genome formula’ by associating a relative copy number to each genomic segment. Thus, when applied to the FBNSV infecting V. faba plants under the experimental conditions shown in Fig. 1 , the genome formula is 3 C 3 M 13 N 2 R 1 S 7 U1 10 U2 16 U4 , where numbers indicate the median copy number of each segment, rounded to the nearest integer, relative to that of the least abundant segment, and superscript letters indicate the name of the segment. The use of mean frequency values (instead of median) gives a very similar genome formula. It must be noted, however, that some segments are dispensable for infection under laboratory conditions (see Methods for details) and that they can occasionally be lost upon artificial agroinoculation of plants [13] , [14] . Hence, we prefer the use of median values because they are less affected by these occasional segment losses than is the mean. As all the results presented in this report were obtained with total viral DNA extracted from infected plant tissues, we assessed whether the estimated genome formula was similar for DNA encapsidated into virus particles. In independent plant sets, we compared the relative frequency of segments in total versus encapsidated DNA extracted from the same leaf samples (see Methods ). The results shown in Supplementary Fig. S1 demonstrate that the genome formula in total DNA extractions closely reflects that in encapsidated DNA. The genome formula does not depend on initial conditions We first tested whether the genome formula in systemically infected plants depends on the initial frequency of the respective segments at inoculation. For this, we prepared two inocula with different segment proportions. 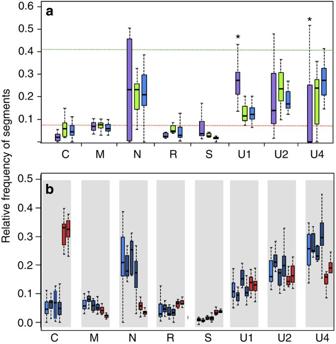Figure 2: Factors affecting the genome formula of FBNSV. (a) The relative frequency of segment S (S++, purple) or segment C (C++, green) was increased fivefold in the inocula. The resulting frequencies in the uppermost leaf of infected plants are summarized in the box-plots (black bar is the median and vertical dotted line delineates 1.5 times the distance between the 25th and 75th percentile of the distribution). For comparison, data from Vf-Agr1, Vf-Agr2 and Vf-Agr3 (Fig. 1) were pooled and plotted in blue. The number (n) of infected plants analysed in each set isn=12 andn=7 for S++ and C++, respectively. The upper green dotted line indicates the frequency of S or C in the inoculum, whereas the lower dotted red line indicates the frequency of all other segments. Between plant sets, significant differences (*) were detected by an analysis of variance (ANOVA) test (plant set effect on the frequency of U1 and U4:F1, 27=33 and 9.04,P-values=3.6 × 10−6and 0.0045, respectively). (b) The relative frequency of FBNSV segments inV. fabaplants inoculated by aphids is plotted in dark blue and compared with that in agro-inoculated plants (light blue on the left, same Vf-Agr1-3 data as ina). Three-independent aphid inoculation experiments named Vf-At1 (n=10), Vf-At2 (n=6) and Vf-At3 (n=32) are, respectively, plotted from left to right. The frequency of the segments was not affected by the mode of inoculation, as demonstrated by ANOVA tests detailed inSupplementary Table S2. The segments’ frequency inM. truncatulaplants inoculated by aphid was estimated in two plant sets, Mt-At1 (right,n=12) and Mt-At2 (left,n=13), and is plotted in red. The host species had a significant effect on all segments except U1, as shown by ANOVA tests detailed inSupplementary Table S4. The genome formulae of FBNSV inV. faba(GFVf) and inM. truncatula(GFMt) were calculated by pooling all Vf-At and Mt-At data sets, respectively, and are markedly distinct: GFVf=3C3M9N2R1S6U111U215U4and GFMt=12C1M1N2R2S5U16U27U4. Figure 2a shows the results of two-independent plant sets infected with either a fivefold excess of segment S (S++) or of segment C (C++). As previously, the uppermost leaf level was analysed for each plant set when the infection had developed fully and provoked the arrest of plant growth. The frequency of the different FBNSV segments in these two plant sets proved very similar to that in plants inoculated with equal quantities of all segments. The only significant differences detected were for segments U1 and U4 in set S++ ( Fig. 2a ). The very low median frequency observed for segment U4 in the plant set S++ is due to the 9 out of 12 plants where segment U4 was lost at inoculation—a situation sometimes observed when segments that are dispensable for infection under laboratory conditions are inoculated at too low a frequency. In the C++ set, only 2 out of 7 plants had lost U4. Figure 2: Factors affecting the genome formula of FBNSV. ( a ) The relative frequency of segment S (S++, purple) or segment C (C++, green) was increased fivefold in the inocula. The resulting frequencies in the uppermost leaf of infected plants are summarized in the box-plots (black bar is the median and vertical dotted line delineates 1.5 times the distance between the 25th and 75th percentile of the distribution). For comparison, data from Vf-Agr1, Vf-Agr2 and Vf-Agr3 ( Fig. 1 ) were pooled and plotted in blue. The number ( n ) of infected plants analysed in each set is n =12 and n =7 for S++ and C++, respectively. The upper green dotted line indicates the frequency of S or C in the inoculum, whereas the lower dotted red line indicates the frequency of all other segments. Between plant sets, significant differences (*) were detected by an analysis of variance (ANOVA) test (plant set effect on the frequency of U1 and U4: F 1, 27 =33 and 9.04, P -values=3.6 × 10 −6 and 0.0045, respectively). ( b ) The relative frequency of FBNSV segments in V. faba plants inoculated by aphids is plotted in dark blue and compared with that in agro-inoculated plants (light blue on the left, same Vf-Agr1-3 data as in a ). Three-independent aphid inoculation experiments named Vf-At1 ( n =10), Vf-At2 ( n =6) and Vf-At3 ( n =32) are, respectively, plotted from left to right. The frequency of the segments was not affected by the mode of inoculation, as demonstrated by ANOVA tests detailed in Supplementary Table S2 . The segments’ frequency in M. truncatula plants inoculated by aphid was estimated in two plant sets, Mt-At1 (right, n =12) and Mt-At2 (left, n =13), and is plotted in red. The host species had a significant effect on all segments except U1, as shown by ANOVA tests detailed in Supplementary Table S4 . The genome formulae of FBNSV in V. faba (GF Vf ) and in M. truncatula (GF Mt ) were calculated by pooling all Vf-At and Mt-At data sets, respectively, and are markedly distinct: GF Vf =3 C 3 M 9 N 2 R 1 S 6 U1 11 U2 15 U4 and GF Mt =12 C 1 M 1 N 2 R 2 S 5 U1 6 U2 7 U4 . Full size image To further assess whether inoculation mode could affect the genome formula of FBNSV establishing in V. faba , we switched from agro-inoculation to aphid transmission, that is, the natural transmission mode. We fed aphids for 3 days on four, randomly chosen, infected plants. Aphids were then pooled, and used to inoculate young test plants for another 3-day period (five aphids per test plant). Four weeks later, when plants showed symptoms of systemic infection and stopped developing new leaves, the uppermost leaf level was analysed by Q-PCR. The results of three-independent replicates of the experiment (noted as Vf-At1, Vf-At2 and Vf-At3 in Fig. 2b ) show that the FBNSV genome formula obtained after aphid inoculation is close to that obtained after agro-inoculation ( cf. genome formulae in V. faba in Figs 1 and 2b ). Whatever the segment considered, no significant frequency difference could be detected when comparing the two modes of inoculation ( Fig. 2b and Supplementary Table S2 ). Altogether, these results demonstrate that the various segments of the FBNSV genome reproducibly adjust to a specific relative frequency during systemic invasion of the host plant V. faba , whatever the initial conditions at inoculation. We propose to refer to these adjusted frequencies of the different segments as the ‘setpoint genome formula’. The genome formula converges on a setpoint An intriguing observation from Figs 1 and 2 is the large variance in segment frequencies observed among individual plants within all plant sets but around one single-dominant situation. We further used the plant set with the highest number of infected plants, that is, the set Vf-At3 inoculated by aphids ( Fig. 2b ), to assess a possible temporal evolution of the genetic composition of within-host FBNSV populations. In this set, the plants were all inoculated at the second leaf stage but had their development arrested by virus infection at either the 5th ( n =2), 6th ( n =16), 7th ( n =10) or 8th ( n =4) leaf stage, suggesting potentially different kinetics of infection in different plants. To compare plants within a homogeneous sub-set, we focused on the 16 plants whose development was arrested at the six-leaf stage. As leaves appear consecutively during the development of viral disease until full appearance of symptoms provokes plant development arrest, lower leaves are likely to have been colonized by the virus earlier than upper leaves. A time series of the genetic structure of the virus population could thus be reconstituted by comparing the segment frequencies in the six successive leaf levels. 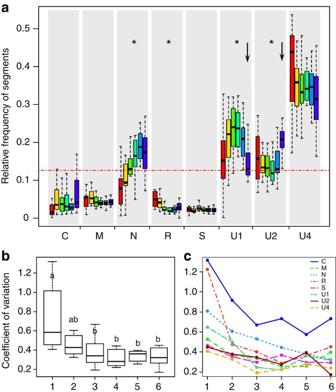Figure 3: Convergence of FBNSV within-host populations to the setpoint genome formula. (a) The frequency of all FBNSV segments was analysed in 16 plants from Vf-At3 set (plant set used inFig. 2b), which developed six leaf levels before the virus induced developmental arrest. For each box plot, the horizontal black bar represents the median of the distribution and the vertical dotted line delineates 1.5 times the distance between the 25th and 75th percentile of the distribution. For each segment, the results from leaf levels 1 to 6 are represented in different colours from left to right. The segments indicated with an asterisk accumulated at different frequency in different leaf levels (see analysis of variance (ANOVA) tests of the effect of leaf-levels for each of the eight segments inSupplementary Table S3). However, only the median frequency of U1 and U2 was still changing significantly at later stages of infection, between leaf 4 and leaf 6 (black arrows, Tukey HSD pair test,P-values=0.014 and 0.00041, respectively). (b) Each box-plot represents the distribution of the coefficients of variation (CV) of the eight segments in a given leaf level among plants. The significant differences among leaf levels was confirmed by an ANOVA test:F5, 41=4.19,P-values=0.0036. Letters indicate significant differences between leaf levels, which were estimated by Tukey HSD pair tests (P-value between leaf levels 1–3, 1–4, 1–5 and 1–6=0.017, 0.0086, 0.049, 0.046, respectively). Black bars within box plots represent medians and vertical dotted lines delineate 1.5 times the distance between the 25th and 75th percentile of the distribution. (c) In successive leaf levels noted on thexaxis, changes of the CV of each segment are represented by different coloured lines as indicated. Figure 3a shows that the median frequency did not change significantly across leaf levels for segments C, M, S and U4 ( Fig. 3a and Supplementary Table S3 ), whereas N and R stabilized at leaf level 4, and only segments U1 and U2 were still significantly changing at later stages of infection (between leaf levels 4 and 6, Fig. 3a ). This observation suggests that the median genome formula within a plant set stabilizes rapidly around the setpoint formula during disease progression. Figure 3: Convergence of FBNSV within-host populations to the setpoint genome formula. ( a ) The frequency of all FBNSV segments was analysed in 16 plants from Vf-At3 set (plant set used in Fig. 2b ), which developed six leaf levels before the virus induced developmental arrest. For each box plot, the horizontal black bar represents the median of the distribution and the vertical dotted line delineates 1.5 times the distance between the 25th and 75th percentile of the distribution. For each segment, the results from leaf levels 1 to 6 are represented in different colours from left to right. The segments indicated with an asterisk accumulated at different frequency in different leaf levels (see analysis of variance (ANOVA) tests of the effect of leaf-levels for each of the eight segments in Supplementary Table S3 ). However, only the median frequency of U1 and U2 was still changing significantly at later stages of infection, between leaf 4 and leaf 6 (black arrows, Tukey HSD pair test, P -values=0.014 and 0.00041, respectively). ( b ) Each box-plot represents the distribution of the coefficients of variation (CV) of the eight segments in a given leaf level among plants. The significant differences among leaf levels was confirmed by an ANOVA test: F 5, 41 =4.19, P -values=0.0036. Letters indicate significant differences between leaf levels, which were estimated by Tukey HSD pair tests ( P -value between leaf levels 1–3, 1–4, 1–5 and 1–6=0.017, 0.0086, 0.049, 0.046, respectively). Black bars within box plots represent medians and vertical dotted lines delineate 1.5 times the distance between the 25th and 75th percentile of the distribution. ( c ) In successive leaf levels noted on the x axis, changes of the CV of each segment are represented by different coloured lines as indicated. Full size image An interesting follow-up question is whether the observed fluctuations of segment frequencies around the median values are maintained over time, or whether FBNSV populations within each individual plant tend to converge to the setpoint genome formula. In the same plant set as in Fig. 3a , we calculated the coefficient of variation of the frequency of all eight segments and found that it decreased significantly from lower to upper leaf levels ( Fig. 3b ). Noticeably, the same pattern could be observed for each individual segment ( Fig. 3c ), suggesting that all are submitted to frequency-dependent selection. Frequency co-variation was detected in only 2 out of 28 possible pairs of segments (C-U1 and N-U4) in the data set presented in Fig. 3 (Spearman’s rank correlation, for P -values for all pair wise combinations, see Supplementary Table S4 ), suggesting the absence of one major regulatory segment that would control the frequency of others. The genome formula may affect virus accumulation and symptoms The previous observations indicate that, under these experimental conditions, the segment frequencies within each plant, and hence across plants, converge towards the setpoint genome formula. We thus asked whether the genome formula has any adaptive significance for FBNSV. To that end, we looked for a possible relationship between the proximity of the FBNSV population to the setpoint genome formula and viral accumulation in planta . In the plant set Vf-At3, both virus accumulation and the distance of FBNSV populations from the setpoint formula were calculated in all leaves of plants with 6, 7 or 8 leaves ( Fig. 4 : blue, red and green lines, respectively). The viral load was calculated simply by summing the Q-PCR estimates of all eight segments (relative to a reference plant gene, see Methods ). The distance to the setpoint genome formula was estimated by summing up the absolute difference between each segment frequency and its specific setpoint formula value [16] (see Methods , distance to the setpoint genome formula (dGF1)). The setpoint genome formula values used here to estimate the distance were calculated by pooling all independent V. faba plant sets shown in Figs 1 , 2 and 3 , except set Vf-At3. 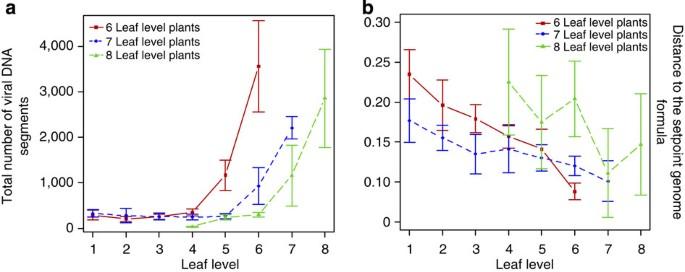Figure 4: Genome formula may impact on viral accumulation and plant development. (a) Viral accumulation was measured in all leaves of plants that developed 6 (red square,n=16), 7 (blue diamond,n=11) or 8 (green triangle,n=4) leaf levels. The scale on the left indicates the total number of DNA circles per leaf-sample accumulated at each leaf level. (b) The distance of FBNSV populations to the setpoint genome formula was calculated in all leaves of plants that developed 6 (red square), 7 (blue diamond) or 8 (green triangle) leaf levels. The scale on the left indicates the distance of FBNSV populations to the genome formula, calculated as described in Methods. Error bars are s.d. Figure 4: Genome formula may impact on viral accumulation and plant development. ( a ) Viral accumulation was measured in all leaves of plants that developed 6 (red square, n =16), 7 (blue diamond, n =11) or 8 (green triangle, n =4) leaf levels. The scale on the left indicates the total number of DNA circles per leaf-sample accumulated at each leaf level. ( b ) The distance of FBNSV populations to the setpoint genome formula was calculated in all leaves of plants that developed 6 (red square), 7 (blue diamond) or 8 (green triangle) leaf levels. The scale on the left indicates the distance of FBNSV populations to the genome formula, calculated as described in Methods. Error bars are s.d. Full size image In the three sub-sets where plants developed 6, 7 or 8 leaves, respectively, before arresting development, several observations suggest a causal link between the distance of FBNSV populations to the setpoint genome formula, the rapid increase in viral load, and the inhibition of plant development: (i) in all plant subsets (all three curves: green, red and blue), the distance of the infecting FBNSV populations to the V. faba setpoint genome formula decreased monotonically as infection progressed ( Fig. 4b ), implying that, within each plant, the FBNSV population evolved continuously towards the setpoint formula; (ii) viral accumulation increased with time, as seen by leaf level ( Fig. 4a ); (iii) viral accumulation rose earlier in plant sets where the distance to the genome formula reached its lowest value more rapidly; and (iv) viral accumulation rose earlier in plant sets where development was arrested earlier ( Fig. 4a ). In an alternative calculation, where the distance to the setpoint formula was weighted for all segments as the proportional deviation from the setpoint value (see dGF2 in Methods), the pattern observed in Fig. 4b was not qualitatively affected ( Supplementary Fig. S2 ). A direct correlation between viral accumulation and distance to the setpoint genome formula could not be detected in individual leaves of a comparable leaf level in the plant set Vf-At3 (Spearman’s rank correlation coefficient at leaf level 4, 5 or 6: P -values=0.087, 0.57, 0.97, respectively). Possible reasons for this are discussed below. The setpoint genome formula of FBNSV is host-dependent Finally, in order to test for a possible host effect on the setpoint genome formula, we used the aphid inoculation procedure described above to transmit FBNSV from infected V. faba plants to a set of plantlets of the related legume species Medicago truncatula . Symptoms of leaf yellowing and curling revealed the success of systemic infection within 10–25 days post-inoculation but, in contrast to the situation observed in V. faba , persistent FBNSV infection did not inhibit growth and new leaf development in M. truncatula . Four weeks post-inoculation, whole leaflets were collected from the uppermost leaf level of each infected M. truncatula plant and processed for Q-PCR analysis of viral segment frequencies as above (for easy comparison, these results are shown in red in Fig. 2b ). The experiment was repeated twice using different infected V. faba source plants, different aphid cohorts and different M. truncatula plantlets ( Fig. 2b Mt-At1 and Mt-At2), and consistently demonstrated an effect of the host on the genetic structure of FBNSV populations. Except for U1, all genome segments accumulated at significantly different frequencies in the two host species ( Fig. 2b and Supplementary Table S5 ). This resulted in markedly distinct setpoint genome formulae in M. truncatula (12 C 1 M 1 N 2 R 2 S 5 U1 6 U2 7 U4 ) and in V. faba (3 C 3 M 9 N 2 R 1 S 6 U1 11 U2 15 U4 ), where the largest differences pertained to segments C, N and U4. In all organisms, gene expression is regulated through various distinct pathways, including transcriptional and post-transcriptional regulation of mRNAs, as well as translational control and post-translational modification of proteins. Upstream of all these mechanisms, the regulatory role of the actual gene copy number (GCN) is becoming increasingly recognized. The GCN, and changes thereof (that is, copy number variation), of specific genes present within individual cells is thought to greatly affect gene expression in most (if not all) organisms [17] , [18] . For example, copy number variation has been associated with both control of development and genetic disease in organisms ranging from humans [19] to insects [20] , and with stress adaptation processed in protozoa [21] and bacteria [18] . The hijacking of host regulatory processes to fine-tune viral infection cycles is well known and has received enormous attention [22] , [23] , [24] , [25] , [26] , [27] . However, despite increasing evidence that copy number variation is a key regulatory process [28] , its potential exploitation by viruses has not been explored to date. This is particularly surprising given the ubiquitous impact of GCN on phenotypic expression [28] , on population genetics and evolution [29] , and when considering the enormous potential of such regulation in the diverse genome structures and expression strategies of viruses. We believe that regulation of GCN might explain the establishment of a setpoint genome formula of FBNSV during systemic host infection. The mechanism actually driving adjustment of FBNSV populations to the setpoint genome formula in a given host remains enigmatic. A hypothesis (H1) that fits our results postulates both stochastic events at the segment (gene) level, and positive selection at the system (genome) level: at early steps of the plant infection, different cells could be infected by distinct ensembles of virus particles, among which the relative frequency of each segment would vary randomly (particularly if the number of particles infecting each individual cell is relatively small). Infecting ensembles with relative segment frequencies resulting in higher replication would produce more offspring. In such a scenario, if the eight FBNSV genome segments were replicated at the same rate and have similar chances to be transmitted to new cells, the pattern of relative segment frequencies established in newly infected tissues should reflect that from cells producing more viral offspring, and should thus progressively adjust to and stabilize at the genome formula maximizing replication in a given environment. It seems reasonable to assume that the different segments have the same replication efficiency, because they are similar in length (980–1,003 nucleotides) and all harbour a conserved origin of replication interacting with the same viral ‘replication factor’ (REP) encoded by segment R [13] . Likewise, once individually encapsidated (or associated) with the same coat protein (encoded by segment S), all segments can move similarly through plasmodesmata, and can thus exit the cell, and enter sieve elements or adjacent uninfected cells. Hypothesis H1 is supported partially by the results described in Figs 3 and 4 . Indeed, numerous FBNSV populations in individual V. faba plants converge to the same genome formula, suggesting selection of a specific relative frequency of genome segments in a given environment. Moreover, the viral load within leaves increased in parallel to adjustment of the population around the setpoint genome formula, possibly revealing a link between the two phenomena. Not all our results, however, reflect this causal link between the distance of FBNSV populations to the setpoint genome formula (as calculated here) and viral load. Specifically, there are two such observations: (i) we detected no significant correlation between viral load and distance to the setpoint genome formula within comparable leaf levels of our plant sets and (ii) plants in which development was arrested at seven leaves were initially closer to the setpoint formula than those in which development was arrested at six leaves ( Fig. 4b ), yet convergence to the setpoint formula appeared slower in the former case and the increase in viral load was delayed accordingly. One explanation for this discrepancy may be the very nature of the distance measure we used, which ascribes the same weight to variation in all segments, and assumes a similar effect when a segment is either under- or over-represented. We felt that current knowledge of the FBNSV replication cycle is too fragmentary to justify any other weighting. It is highly unlikely, however, that quantitative variation in relative frequency above or below the setpoint value is strictly equivalent for all segments. It is much more likely that subtle co-variations in the frequency of several segments, yet to be identified, govern the efficiency of viral replication within host cells. We thus believe that our distance calculations only partly capture the effect of segment frequency variation when making comparisons at the stage at which plant development was arrested ( Fig. 4 ), and that important aspects of the dynamics of how viral populations arrive at the point where they achieve high viral loads and eventually arrest plant development (in V. faba ) are still obscure. A simple alternative mechanism to explain adjustments to the genome formula in FBNSV populations could be differences in segment replication rates. Indeed, the sequences of the eight segments diverge considerably, even in non-coding regions [13] , [30] , and a distinct regulation during replication cannot be excluded. Under this hypothesis (H2), the replication rate of each segment would directly reflect the observed differences in accumulated GCNs. The segment-specific replication rate would have been selected to give a constant optimal genome formula and, given the same assumptions as in H1 (viral particles have similar chances to exit and enter cells whatever segment they contain), any initial segment frequency would return rapidly to the endpoint formula. A major caveat of H2 is that segments replicating slowly would be outcompeted rapidly by the others and lost. Our observation is that all segments detected in lower leaf-levels are generally maintained in upper leaf-levels, thus H2 is untenable without invoking additional unknown mechanisms ensuring maintenance of slowly replicating segments. Considering that the genome formula described here applies similarly to encapsidated DNA ( Supplementary Fig. S1 ), a most intriguing question for FBNSV, and multipartite viruses in general [4] , [12] , is that of the number of virus particles entering individual cells. Assuming that the probability for a genome segment to enter an individual cell depends solely on its relative frequency within the population, infection of 95% of susceptible cells by at least one copy of each segment would require the entry of approximately 160 virus particles per cell if the population is at the setpoint genome formula. The multiplicity of cell infection (MOI), defined as the number of virus genomes initiating infection within individual cells, has been estimated for a small number of monopartite virus species infecting animals [31] , [32] , [33] and plants [34] , [35] , [36] to range from 1–13. In most cases, the virus is believed to infect new cells in the form of virus particles, thus connecting the MOI value to the number of particles penetrating each cell, and suggesting that the latter is of the order of a few units to a few tens of units. Genome multi-compartmentalization, augmented by the observed variation in frequency across segments of FBNSV, induces an extra cost at the step of cell infection because the number of virus particles required is one or two orders of magnitude higher. In fact, the required number of particles per cell for FBNSV appears so high that it is tempting to imagine a regulatory mechanism that would group one or more copies of each segment into a reasonably sized infectious unit. Further investigation on how multipartite viruses deal with the acute problem of MOI is clearly required. The dependence of setpoint genome formula on host species opens another avenue for future investigation. On the one hand, one could argue that multipartite viruses are highly polymorphic biological systems, and that the distinct formulae observed in V. faba and in M. truncatula stem simply from a different optimal composition of FBNSV populations in these two hosts, as explained by scenario H1 described above. On the other hand, the different formulae observed in M. truncatula may be suboptimal, and may more trivially reflect mal-adaptation of this isolate of FBNSV to this particular host (the FBNSV isolate used here was isolated originally from V. faba [13] ). As no consensus sequence change could be observed in FBNSV populations after two successive passages in V. faba [30] , longer experimental evolution both in M. truncatula and in V. faba may be required to assess whether the genome formula evolves, and to identify adaptive mutations responsible for the putative formula change. A recent study described the phenomenon of ‘gene-accordion’ in the monopartite vaccinia poxvirus [37] . This latter study demonstrated that, under specific selection pressure, a vaccinia virus gene was amplified rapidly by successive duplications, which expanded the single-molecule genome and was immediately beneficial for the virus. The same authors further demonstrated that, once amplified, one of the copies of the corresponding gene eventually acquired a beneficial mutation decreasing the need for multiple extra copies, which were then progressively eliminated, compacting back the viral genome. Multipartite viruses appear particularly well adapted to the gene-accordion phenomenon, which can be implemented through the plasticity of the genome formula. The immediate change in GCN when FBNSV is transmitted from V. faba to M. truncatula appears as a spectacular illustration of the ease with which multipartite viruses can use gene-accordion, and could illustrate a major advantage of this peculiar genome architecture. Gene or segment copy number regulation is similarly possible for all multipartite viruses, raising the question of the significance of our discovery for viral species other than FBNSV. Although no direct investigation has addressed this question, some data indicating unequal accumulation of different genome segments can be found, for example, in studies on cucumber mosaic virus [38] , [39] , [40] , [41] , tomato aspermy virus [42] , [43] and brome mosaic virus [44] —all positive-sense ssRNA viruses unrelated to FBNSV. These earlier studies were either purely descriptive, analysing the physical and/or chemical properties of the virus particle [38] , [39] , [42] , [44] , or focused on technical developments for RNA quantification [40] , [41] , [44] . Nevertheless, they suggest that the regulation of segment copy number may be a general feature of multipartite viruses. It will be of interest to extend the question of the control of GCN to those segmented viruses encapsidating one copy of each genome segment in a single virus particle [45] . A series of studies on the switch from lytic to lysogenic cycle of the monopartite bacteriophage λ (refs 46 , 47 ) demonstrated that the number of genomes entering a host cell is instrumental in determining the phenotype expressed by the phage, that is, replicate fast and kill the host (lytic), or integrate into the host genome and protect it (lysogenic). So, whether infection is initiated with one or more copies of a monopartite genome can alone decide the fate of both virus and host cell. Focusing on the initial step of cell infection, segmented viruses co-encapsidating one copy of each segment resemble the monopartite situation with an equal copy number of each gene. In contrast, multipartite viruses can potentially adjust the copy number of each segment, even at cell entry. Whether this additional level of regulation at the very first step of infection benefits multipartite viruses is unclear, but it would be precluded by all other types of viral genome organization. The potential benefit of differential control of GCN in segmented and multipartite viruses imposes direct constraints on the frequencies of individual genome segments. This clearly comes at additional cost and thus questions regarding the origin, and reasons for the evolution, of such biological systems deserve to be revisited in the light of the results described here on FBNSV. Virus isolate and inoculation The isolate of FBNSV used in this study was originally isolated from V. faba in Ethiopia [13] . From this isolate, agrobacterium-compatible clones of each of the eight FBNSV segments (DNA C, M, N, R, S, U1, U2 and U4) were prepared, and shown to together constitute a fully infectious and transmissible clone of FBNSV [13] . Briefly, Agrobacteria containing tandem repeat clones of each segment were grown in NZY+ medium (0.1% NZ amine, 0.5% yeast extract, 0.5% NaCl, 12.5 mM MgCl 2 , 12.5 mM MgSO 4 and 0.4% glucose at pH 7.5) until an optical density (OD 600 ) of 2–3 was reached. Mixtures of these bacterial suspensions were then prepared in ad hoc proportions, centrifuged and resuspended in 40 ml of MS buffer [48] containing 30 μM of acetosyringone and 1 mM of MES (morpholinoethanesulfonic acid). These mixtures were then needle-inoculated into the stem of 10-day-old V. faba plants at the two-leaf stage, and resulted in infection of around 20% of the inoculated plants. An earlier report demonstrated that the closely related Faba bean necrotic yellow virus (FBNYV) can replicate and progress systemically within its V. faba host plants, under laboratory conditions, when either one of C, N, U2 or U4 is missing [14] . However, how the absence of each of these segments induces differences in the infection kinetics and aphid transmission remains to be characterized in detail for FBNYV and for the FBNSV isolate used here. Despite these observations, and because in all described natural isolates of FBNYV and FBNSV the eight ‘core’ genome segments were always present, all eight are considered to be integral parts of the viral genome [30] . Plant growth conditions Broad bean (V. faba, var. ‘Sevilla’ from Vilmorin) and M. truncatula (Jemalong A17) plants were grown in soil treated with Trigard 5 W (2 g per 5 l) in a growth chamber with a 13/11 h day/night photoperiod, a temperature of 26/20 °C day/night and 70% hygrometry within an S2 restricted-access confinement facility. Aphid growth conditions The Acyrthosiphon pisum colony was maintained on V. faba plants in environmental growth chambers at a temperature of 23/21 °C and a photoperiod of 13/11 h (day/night), ensuring reproduction through parthenogenesis. Cohorts of aphids were allowed a 3-day acquisition period on V. faba plants infected by FBNSV for 30 days (30 dpi). Then, aphids were transferred to 10-day-old V. faba plantlets, or on M. truncatula at the three-leaf stage, and allowed an inoculation period of three additional days. Aphids were finally killed by spraying the young test plants with Pirimor G (1 g l −1 in water). Whether agro-inoculation or aphid-transmission was used, symptoms of systemic infection appeared on newly developed leaves between 10 and 25 dpi, as inward leaf-curling and yellowing. The apical growth in V. faba plants was totally inhibited shortly after systemic symptoms appeared, but the plants survived for several additional weeks. Similar symptoms appeared on M. truncatula leaves between 10 and 25 dpi, but the viral infection did not stop apical development in this species and symptomatic plants continued growing indefinitely. DNA extraction and Q-PCR conditions One V. faba leaflet per leaf level of symptomatic plants was punched four times on the main vein to collect four leaf disks (6-mm φ each), except for the youngest leaf level for which one entire leaflet was harvested. Concerning M. truncatula, one leaflet per leaf level was harvested and analysed. Sampling was carried out between 30 and 35 dpi for both V. faba and M. truncatula . Total DNA from these samples was extracted according to a modified Edwards protocol [49] with an additional washing step with 70% ethanol. DNA was resuspended with 200 μl of water, and 10-fold diluted samples were used for Q-PCR. For extracting encapsidated DNA, the leaf disks were ground in 400 μl of a mild extraction buffer (200 mM Tris HCl, 250 mM NaCl, 1 mM PVP-40, 0.05% Tween 20) described earlier [50] . Samples were vortexed and then clarified for 5 min at 10,000 g. To remove all unencapsidated DNA, samples were incubated with one volume of nucleic acid-digestion solution (200 mM Tris-HCl, 1 mg ml −1 DNase I, 1 mg ml −1 RNase A) for 30 min. at 37 °C. After addition of 5 mM EDTA, 0.2% SDS and 2 mg ml −1 proteinase K (final concentrations) and further incubation for 30 min, the proteinase K was denatured by heating samples at 95 °C for 15 min. DNA was finally precipitated with isopropanol, resuspended in water and stored at −20 °C until use for Q-PCR. In these samples, no plant DNA (tested with V. faba legumin B gene LeB4 , GenBank accession Nb X03677 ) could be Q-PCR-amplified, controlling for the efficient elimination of unprotected (unencapsidated) DNA. All Q-PCR reactions (40 cycles of 95 °C for 10 s, 63 °C for 10 s and 72 °C for 10 s) were carried out using the LightCycler FastStart DNA Master Plus SYBR green I kit (Roche) in a LightCycler 480 thermocycler (Roche), following the manufacturer’s instructions. The primers ( Supplementary Table S6 ) were used at a final concentration of 0.3 μM. In each PCR plate, fluorescence data were normalized with a calibrated reference sample for each segment (one of the plasmid dilutions initially used to establish standard curves), and analysed with the LinRegPCR program [51] . Relative frequencies were then calculated in each sample by dividing the estimated number of DNA copies of a given segment by the sum of the number of copies of all eight segments. To determine overall viral accumulation, the sum of the estimated number of copies of each segment was divided by that of a host plant gene ( V. faba legumin B gene LeB4 , GenBank accession Nb X03677 ), normalizing the amount of plant material analysed in all samples. Statistical analysis All statistical tests were carried out with the R and JMP softwares (R Development Core Team, 2011, version 2.12.0; JMP10). The nature and results of each statistical test are indicated in the Results, figure legends and Supplementary Tables . For analysis of variance tests, we used fixed- or mixed-effect models for analysing differences in the frequency of the segments, or differences in their coefficient of variation, depending on the nature of the segment, the experimental replicate, the conditions at inoculation or the leaf level. Whenever several leaf-levels were analysed in the same plant set (that is, repeated measures in the same individuals), the plant effect was included in the model as a random effect. The dGF in each sample was calculated as dGF1=∑ 8 i =1 | p i −pf i |/2 according to Manly (eq. 5.7 p. 68) [16] , or alternatively dGF2=∑ 8 i =1 | p i −pf i |/pf i , where i is the segment, p is the relative frequency of the segment in the sample and pf is the relative frequency of the segment in the setpoint genome formula. How to cite this article: Sicard, A. et al . Gene copy number is differentially regulated in a multipartite virus. Nat. Commun. 4:2248 doi: 10.1038/ncomms3248 (2013).